Crystal structure of theAlcanivorax borkumensisYdaH transporter reveals an unusual topology The potential of the folic acid biosynthesis pathway as a target for the development of antibiotics has been clinically validated. However, many pathogens have developed resistance to these antibiotics, prompting a re-evaluation of potential drug targets within the pathway. The ydaH gene of Alcanivorax borkumensis encodes an integral membrane protein of the AbgT family of transporters for which no structural information was available. Here we report the crystal structure of A. borkumensis YdaH, revealing a dimeric molecule with an architecture distinct from other families of transporters. YdaH is a bowl-shaped dimer with a solvent-filled basin extending from the cytoplasm to halfway across the membrane bilayer. Each subunit of the transporter contains nine transmembrane helices and two hairpins that suggest a plausible pathway for substrate transport. Further analyses also suggest that YdaH could act as an antibiotic efflux pump and mediate bacterial resistance to sulfonamide antimetabolite drugs. All cells, both prokaryotic and eukaryotic, require folic acid for the biosynthesis of a diverse range of cellular components. Folic acid is of particular importance in aiding cell growth and division. While the cellular requirement for folates is universal, methods to acquire them vary between prokaryotes and eukaryotes. For example, mammals cannot make folates themselves. Instead, they rely on active transport systems, utilizing membrane-associated folate transport proteins to import this essential vitamin [1] . In plants and most microorganisms, folates must be synthesized de novo through the folate biosynthetic pathway [2] . Because of the presence of this pathway in pathogenic bacteria and its absence in mammals, the folate biosynthetic pathway has been an attractive target for the design of novel antimicrobial drugs. The process of de novo synthesis of folates in bacteria can be simply interpreted as chemically linking pterin, p -aminobenzoic acid (PABA) and glutamic acid together. In Escherichia coli , mutations or deletions of enzymes in the folate pathway are known to generate non-viable phenotypes [3] . The possibility of targeting the folate biosynthesis system for antimicrobial therapeutics was proposed several decades ago based on the observation that sulfonamides prevented bacteria from using the metabolite PABA for folate biosynthesis [4] . Indeed, as early as the 1930s, sulfonamides were widely used as synthetic antibiotics to treat infections caused by a variety of pathogenic bacteria, including Neisseria meningitidis and Pneumococcal pneumonia [5] , [6] . Because of the rapid adaption of bacterial pathogens to antimicrobials, drug resistance to currently administered antibiotics is a serious problem that is rising at an alarming rate. For instance, it only took 2 years for N. meningitidis to develop resistant strains following the introduction of sulfonamides [7] . The problem is of particular severity in treating the parasitic malaria disease. A strong correlation has been found between mutations in Plasmodum falciparum and resistance to sulfonamides [8] , [9] , [10] . The initial identification of enzymes involved in folate biosynthesis was largely carried out in the 1960–70s, leading to the detailed description of this enzymatic pathway [11] , [12] , [13] , [14] , [15] , [16] . However, recent work demonstrated that E. coli AbgT [17] , [18] is capable of catalysing the uptake of the catabolite p -aminobenzoyl-glutamate for de novo folic acid synthesis [18] . Because of this finding, it is hypothesized that AbgT-family transporters [19] contribute to the bacterial folate synthesis pathway by importing p -aminobenzoyl-glutamate for producing this essential vitamin. On the other hand, it has been observed that N. gonorrhoeae MtrF [20] , [21] , also belonging to the AbgT family, functions as an antimicrobial resistance protein. It is needed for the high-level resistance of gonococci to hydrophobic antimicrobials [20] , [21] . To date, ∼ 13,000 putative transporters of the AbgT family have been identified. However, among proteins in this diverse family, only E. coli AbgT [17] , [18] and N. gonorrhoeae MtrF [20] , [21] have been partially characterized. Thus far, there is no structural information available for this family of membrane proteins. In A. borkumensis , the gene ydaH [22] encodes a membrane protein YdaH of previously unknown structure and function. Alignment of protein sequences suggests that this protein belongs to the AbgT family of transporters [19] . To understand how members of the AbgT family work, we here present the crystal structure of YdaH, revealing a novel topology distinct from other families of transporters. Here we show that YdaH is capable of exporting the folate metabolite PABA from bacterial cells. A combination of the three-dimensional structure and genetic analysis allows us to identify important residues for the function of this membrane protein. Our data suggest that A. borkumensis YdaH could function as an antibiotic efflux pump and remove sulfonamides from the cell to mediate bacterial resistance to this class of antimetabolites. Overall structure of A. borkumensis YdaH A. borkumensis YdaH consists of 492 amino acids, sharing 34% sequence identity with E. coli AbgT ( Supplementary Fig. 1 ). The crystal structure of YdaH was determined to a resolution of 2.96 Å ( Fig. 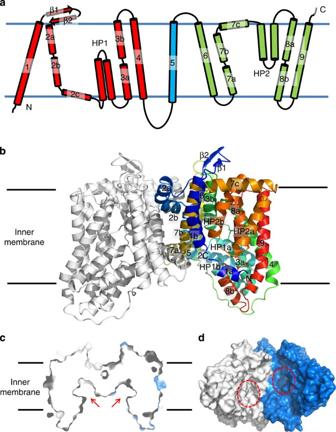Figure 1: Structure of theA. borkumensisYdaH transporter. (a) Transmembrane topology ofA. borkumensisYdaH. The transporter contains nine transmembrane helices (TMs) and two hairpins (HPs). (b) Ribbon diagram of a dimer of YdaH viewed in the membrane plane. The right subunit of the dimer is coloured using a rainbow gradient from the N terminus (blue) to the C terminus (red), whereas the left subunit is coloured grey. The YdaH dimer forms a bowl-shaped structure with a concave aqueous basin facing the intracellular solution. (c) Surface representation of the YdaH dimer sliced through the middle of the protein. Each protomer forms an internal cavity (red arrow), which is accessible to the cytoplasm. (d) Bottom view of a surface representation of the YdaH dimer, indicating a solvent accessible cavity (red circle) from each protomer of the protein. The two protomers are coloured gray and blue. 1 and Table 1 ). Four molecules of YdaH were found in the asymmetric unit, forming two independent assembled dimers ( Supplementary Fig. 2 ). Superimposition of these two dimers gives a root mean squared deviation of 1.0 Å (942 Cα atoms; Supplementary Fig. 3 ), suggesting that their conformations are nearly identical to each other. The dimeric form of YdaH in the crystal lattice is also in good agreement with the oligomerization state of this membrane protein in solution where it assembles as a dimer ( Supplementary Fig. 4 ). The topology of YdaH is unique among all known transporters ( Fig. 1a ). The YdaH dimer is bowl shaped with a concave aqueous basin facing the intracellular solution. Viewed in parallel to the membrane, the dimer is about 60 Å tall, 80 Å wide and 60 Å thick, with the transmembrane portion of the transporter lying approximately in the middle ( Fig. 1b ). Thus, the transporter protrudes about 10 Å from each side of the membrane. The rim of the basin is as large as 50 Å. The bowl-shaped structure is 20 Å in depth and deeply penetrates into the inner leaflet of the cytoplasmic membrane. This basin probably allows the aqueous solution to reach the midpoint of the membrane bilayer. It is interesting to note that our crystal structure of YdaH is in good agreement with the predicted topology of E. coli AbgT that the carboxyl (C)-terminal end of this transporter is located at the periplasm [23] . Figure 1: Structure of the A. borkumensis YdaH transporter. ( a ) Transmembrane topology of A. borkumensis YdaH. The transporter contains nine transmembrane helices (TMs) and two hairpins (HPs). ( b ) Ribbon diagram of a dimer of YdaH viewed in the membrane plane. The right subunit of the dimer is coloured using a rainbow gradient from the N terminus (blue) to the C terminus (red), whereas the left subunit is coloured grey. The YdaH dimer forms a bowl-shaped structure with a concave aqueous basin facing the intracellular solution. ( c ) Surface representation of the YdaH dimer sliced through the middle of the protein. Each protomer forms an internal cavity (red arrow), which is accessible to the cytoplasm. ( d ) Bottom view of a surface representation of the YdaH dimer, indicating a solvent accessible cavity (red circle) from each protomer of the protein. The two protomers are coloured gray and blue. Full size image Table 1 Data collection, phasing and structural refinement statistics. Full size table Each protomer of YdaH in the dimer contains nine transmembrane helices (TMs 1–9 and TMs 1′-9′, respectively) and two helical hairpins (HPs 1–2 and HPs 1′–2′, respectively; Fig. 1a and Supplementary Fig. 1 ). The TMs and HPs are designated numerically from the N- to C-termini: TM1 (21–42), TM2 (a (63–79), b (83–99) and c (101–112)), HP1 (a (115–131) and b (135–151)), TM3 (a (155–168) and b (178–194)), TM4 (204–228), TM5 (250–272), TM6 (290–314), TM7 (a (320–334), b (336–354) and c (356–371)), HP2 (a (375–392) and b (396–414)), TM8 (a (418–432) and b (441–452)) and TM9 (458–486). Of the nine TMs, four (TM2, TM3, TM7 and TM8) are broken into segments within the membrane. In addition, the helices making up HPs 1 and 2 are relatively short and can only span a portion of the inner membrane. Interestingly, the intramembrane loops of several of these TMs and HPs are right next to one another, allowing the protein to form an internal cavity within the membrane ( Fig. 1c,d ). The YdaH protomer also possesses a relatively small periplasmic domain formed by two loops, between TM1 and TM2 and between TM5 and TM6, respectively. The loop between TM1 and TM2 is found to form two β-strands (β1 and β2), which appear to run antiparallel against one another. In the cytoplasmic region, there is a relatively long loop of 22 residues. This loop connects TM4 and TM5, forming a small cytoplasmic domain of the protomer. The structure of the YdaH dimer can be roughly divided into two cores ( Fig. 2a ). The inner core contains TMs 1, 2, 5, 6 and 7, whereas the outer core comprises TMs 3, 4, 8, 9 as well as HPs 1 and 2. Viewed along the membrane normal, TMs 2a, 2b, 7a and 7b as well as the amino (N)-terminal ends of TMs 1 and 6 form a distinct dimerization domain of the transporter. In particular, TM2a (as well as TM2a′) crosses over to the next subunit, securing the formation of this dimer. Each YdaH protomer shares a substantial intersubunit interface, with an area of ∼ 2,000 Å 2 per protomer. The residues lining the dimerization motif are predominantly hydrophobic in nature. 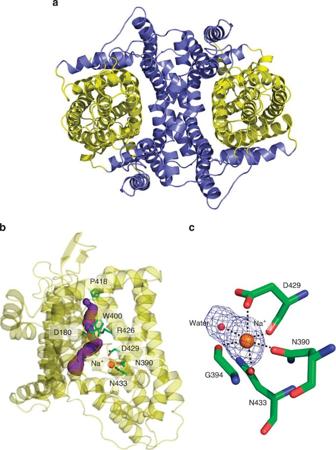Figure 2: Inner and outer cores of YdaH. (a) The inner core of YdaH, comprising TMs 1, 2, 5, 6 and 7 (coloured slate), contributes to dimerization as well as formation of a frame-like structure housing the outer core of the protomer. The outer core of YdaH is composed of TMs 3, 4, 8, 9 as well as HPs 1 and 2 (coloured yellow). (b) The outer core of YdaH forms a channel (coloured purple) spanning approximately from the middle of the inner membrane up to the periplasmic space. This channel was calculated using the programme CAVER (http://loschmidt.chemi.muni.cz/caver). The secondary structural elements of the YdaH protomer are in yellow. Residues D180, N390, W400, P418, R426, D429 and N433 are in green sticks. The bound sodium ion is shown as an orange sphere. (c) The bound Na+(orange sphere) is found to coordinate with N390, G394, D429, N433 and a water molecule (red sphere). The Fo–Fcmap, showing the bound Na+and H2O, is contoured at 3.0σ(blue mesh). Figure 2: Inner and outer cores of YdaH. ( a ) The inner core of YdaH, comprising TMs 1, 2, 5, 6 and 7 (coloured slate), contributes to dimerization as well as formation of a frame-like structure housing the outer core of the protomer. The outer core of YdaH is composed of TMs 3, 4, 8, 9 as well as HPs 1 and 2 (coloured yellow). ( b ) The outer core of YdaH forms a channel (coloured purple) spanning approximately from the middle of the inner membrane up to the periplasmic space. This channel was calculated using the programme CAVER ( http://loschmidt.chemi.muni.cz/caver ). The secondary structural elements of the YdaH protomer are in yellow. Residues D180, N390, W400, P418, R426, D429 and N433 are in green sticks. The bound sodium ion is shown as an orange sphere. ( c ) The bound Na + (orange sphere) is found to coordinate with N390, G394, D429, N433 and a water molecule (red sphere). The F o –F c map, showing the bound Na + and H 2 O, is contoured at 3.0 σ (blue mesh). Full size image While the inner core of the YdaH dimer creates a frame-like architecture, the outer core of each protomer forms a cylindrical structure ( Fig. 2a ). It is most likely that this outer core cylinder forms a substrate-binding site and transport pathway. Interestingly, we found that the outer core cylinder indeed forms a channel spanning approximately from the middle of the inner membrane up to the periplasmic space ( Fig. 2b ). The entrance of this channel is formed by the internal cavity located at the basin of the bowl-shaped structure ( Fig. 1c,d ). This cavity constitutes the loop regions of HP1, HP2, TM3 and TM8 and is accessible to the cytoplasm. On the basis of its location, this internal cavity may form a substrate-binding site of YdaH. Several conserved residues, including D180, W400, P418 and R426, line the wall of the channel ( Fig. 2b ). These residues are expected to play an important role in the function of this transporter. In each protomer of YdaH, a strong spherical electron density sits in the flexible loops between HP2 and TM8. This extra density may come from a trapped water molecule. Because Na + ions were used at all stages of purification and crystallization, it is also possible that the extra electron density originates from a Na + ion. We then used valence calculations [24] to predict if this location can form a metal ion-binding site. The results indicated that this site is most likely Na + specific. Coordinating with this bound Na + ion are the side chains of N390, D429, N433 and the backbone carbonyl oxygens of G394 and D429 ( Fig. 2c ). A water molecule also participates in the interaction, forming another coordinate bond with the Na + ion. YdaH can export p -aminobenzoyl-glutamate As E. coli AbgT has been shown to enable uptake of the folate catabolite p -aminobenzoyl-glutamate, we investigated if the cells expressing YdaH are able to grow on p -aminobenzoyl-glutamate. We made an E. coli -knockout strain BL21(DE3)Δ abgT Δ pabA that lacked the genes abgT [17] , [18] and pabA [25] , which impairs intracellular synthesis of the metabolite PABA. We then expressed the YdaH transporter in this double-knockout strain using the plasmid pET15bΩ ydaH . Surprisingly, the double-knockout BL21(DE3)Δ abgT Δ pabA cells, either transformed with pET15bΩ ydaH or the empty vector pET15b, could not grow in liquid minimal medium (containing 90.4 mM Na 2 HPO 4 , 22.0 mM KH 2 PO 4 , 8.5 mM NaCl, 0.1 mM CaCl 2 , 1.0 mM MgSO 4 , 20.0 mM NH 4 Cl and 22.2 glucose) supplemented with p -aminobenzoyl-glutamate up to 1 μM. Instead, these cells were able to grow in liquid minimal medium when supplemented with 30 nM of the folate metabolite PABA. It should be noted that PABA is capable of diffusing into bacterial cells and participating as an intermediate in the synthesis of the essential folic acid. We thought that YdaH probably could not import p -aminobenzoyl-glutamate as a nutrient for growth. However, this membrane protein may facilitate the transport of PABA across the membrane. Thus, we directly measured the accumulation of PABA in BL21(DE3)Δ abgT Δ pabA expressing YdaH. We compared the radioactive PABA content over time in cells transformed with either pET15bΩ ydaH , encoding A. borkumensis ydaH , or the empty vector pET15b. Surprisingly, the cells expressing YdaH show a significant decrease in the level of [ 3 H]-PABA when compared with cells transformed with the empty pET15b vector ( Fig. 3a ) suggesting that YdaH may act as an efflux pump to export PABA from the cell. 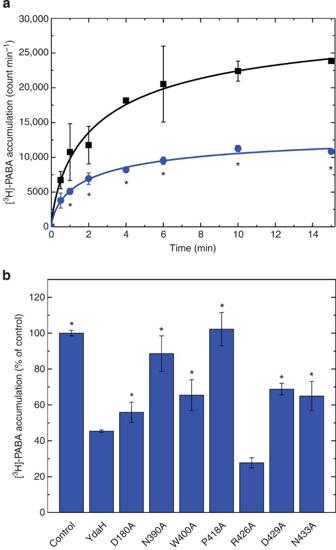Figure 3: Accumulation of radioactive PABA. (a) Time course of [3H]-PABA accumulation byE. coliBL21(DE3)ΔabgTΔpabAdouble-knockout cells transformed with pET15bΩydaHor pET15b. Cells expressingydaH(blue curve) show a significant decrease in [3H]-PABA accumulation when compared with cells carrying the empty vector (black curve). Error bars represent s.d. (n=3). ‘*’ indicates values of BL21(DE3)ΔabgTΔpabA/pET15bΩydaHcells that are significantly different from the control (BL21(DE3)ΔabgTΔpabA/pET15b) values (P<0.04; Student’st-test). (b) Mutants of the YdaH transporter. Cells possessing the mutant transporter D180A, N390A, W400A, P418A, D429A or N433A show a significant increase in the level of [3H]-PABA accumulations compared with the cells expressing wild-type YdaH. However, the cells expressing R426A are able to decrease the [3H]-PABA concentration when compared with cells carrying wild-type YdaH. Error bars represent s.d. (n=3). ‘*’ indicates values of BL21(DE3)ΔabgTΔpabA/pET15b and BL21(DE3)ΔabgTΔpabAcells expressing the mutant transporters that are significantly higher than that of BL21(DE3)ΔabgTΔpabA/pET15bΩydaHexpressing wild-type YdaH (P<0.05; Student’st-test). Figure 3: Accumulation of radioactive PABA. ( a ) Time course of [ 3 H]-PABA accumulation by E. coli BL21(DE3)Δ abgT Δ pabA double-knockout cells transformed with pET15bΩ ydaH or pET15b. Cells expressing ydaH (blue curve) show a significant decrease in [ 3 H]-PABA accumulation when compared with cells carrying the empty vector (black curve). Error bars represent s.d. ( n =3). ‘*’ indicates values of BL21(DE3)Δ abgT Δ pabA /pET15bΩ ydaH cells that are significantly different from the control (BL21(DE3)Δ abgT Δ pabA /pET15b) values ( P <0.04; Student’s t -test). ( b ) Mutants of the YdaH transporter. Cells possessing the mutant transporter D180A, N390A, W400A, P418A, D429A or N433A show a significant increase in the level of [ 3 H]-PABA accumulations compared with the cells expressing wild-type YdaH. However, the cells expressing R426A are able to decrease the [ 3 H]-PABA concentration when compared with cells carrying wild-type YdaH. Error bars represent s.d. ( n =3). ‘*’ indicates values of BL21(DE3)Δ abgT Δ pabA /pET15b and BL21(DE3)Δ abgT Δ pabA cells expressing the mutant transporters that are significantly higher than that of BL21(DE3)Δ abgT Δ pabA /pET15bΩ ydaH expressing wild-type YdaH ( P <0.05; Student’s t -test). Full size image To determine whether the conserved YdaH residues D180, W400, P418 and R426 (lining the inner wall of the tunnel formed by each protomer) are important for the function of the transporter, we mutated these residues into alanines, individually ( Supplementary Table 1 ). On the basis of the crystal structure, we found that residues N390, D429 and N433 are involved in coordinating the bound Na + ion. Therefore, these three residues were also replaced by alanines, respectively ( Supplementary Table 1 ). We then expressed these mutant transporters in BL21(DE3)Δ abgT Δ pabA . Western analysis indicated that the expression levels of these mutant transporters were comparable to that of wild-type YdaH ( Supplementary Fig. 5 ). We then measured the accumulation of [ 3 H]-PABA in cells expressing these mutant transporters. The results showed a significant increase in the levels of [ 3 H]-PABA accumulation in cells possessing the mutant transporter D180A, N390A, W400A, P418A, D429A or N433A, when compared with cells expressing wild-type YdaH ( Fig. 3b ). However, the cells expressing R426A indicated a significant decrease in the [ 3 H]-PABA concentration when compared with cells carrying wild-type YdaH ( Fig. 3b ). The data suggest that YdaH may act as an efflux pump and these amino acids seem to be important for the function of the transporter. YdaH can decrease intracellular folic acid concentration We hypothesized that YdaH is capable of catalysing the efflux of PABA and related compounds. If this is the case, then the cells expressing YdaH may contain a lower level of folic acid content. Therefore, we decided to measure the intracellular folic acid concentration microbiologically using Lactobacillus casei [26] . Cells transformed with pET15bΩ ydaH or pET15b were grown in liquid minimal medium supplemented with 30 nM PABA and harvested when the optical density (OD 600 nm ) reached 0.5. Cells were then assayed to obtain their folic acid concentrations. Consistent with the results from PABA accumulation, the folic acid concentration in cells expressing YdaH was markedly reduced in comparison with cells transformed with the empty vector ( Fig. 4 ). The data support the idea that YdaH may act as an efflux pump and participate in exporting PABA from the cell. 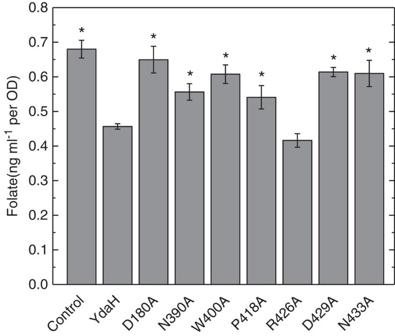Figure 4: Intracellular folic acid concentration. Folic acid concentration inE. coliBL21(DE3)ΔabgTΔpabAdouble-knockout cells expressing YdaH were markedly reduced in comparison with cells transformed with the empty vector. When transformed with plasmid expressing the mutant transporter, D180A, N390, W400A, P418A, D429A and N433A, folic acid production was significantly increased in these cells. However, the level of intracellular folic acid concentration in BL21(DE3)ΔabgTΔpabAcells expressing R426A was nearly identical to that of the double-knockout strain carrying wild-type YdaH. Error bars denote the s.d. of biological replicates,n=4. ‘*’ indicates values of BL21(DE3)ΔabgTΔpabA/pET15b and BL21(DE3)ΔabgTΔpabAcells expressing the mutant transporters that are significantly higher than that of BL21(DE3)ΔabgTΔpabA/pET15bΩydaHexpressing wild-type YdaH (P<0.02; Student’st-test). Figure 4: Intracellular folic acid concentration. Folic acid concentration in E. coli BL21(DE3)Δ abgT Δ pabA double-knockout cells expressing YdaH were markedly reduced in comparison with cells transformed with the empty vector. When transformed with plasmid expressing the mutant transporter, D180A, N390, W400A, P418A, D429A and N433A, folic acid production was significantly increased in these cells. However, the level of intracellular folic acid concentration in BL21(DE3)Δ abgT Δ pabA cells expressing R426A was nearly identical to that of the double-knockout strain carrying wild-type YdaH. Error bars denote the s.d. of biological replicates, n =4. ‘*’ indicates values of BL21(DE3)Δ abgT Δ pabA /pET15b and BL21(DE3)Δ abgT Δ pabA cells expressing the mutant transporters that are significantly higher than that of BL21(DE3)Δ abgT Δ pabA /pET15bΩ ydaH expressing wild-type YdaH ( P <0.02; Student’s t -test). Full size image When transformed with plasmids expressing the mutant transporters D180A, N390A, W400A, P418A, D429A and N433A, folic acid production was significantly increased in these cells. However, the level of intracellular folic acid concentration in cells expressing R426A was nearly identical to that of the double-knockout strain carrying wild-type YdaH ( Fig. 4 ). YdaH may function as an antibiotic efflux pump As PABA is an important precursor for producing essential folic acid in bacteria, we did not understand why the function of YdaH appeared to lower the intracellular PABA concentration. Clearly, there was a significant reduction in PABA content, which led to a decrease in intracellular folic acid concentration in cells expressing the YdaH transporter. We hypothesized that this efflux pump may protect bacterial cells by extruding antimetabolites, such as sulfonamides. Sulfonamides are antimicrobial agents, antimetabolites or growth factor analogues, which specifically inhibit the essential folic acid metabolic pathway in bacterial pathogens. At the chemical level, sulfonamides are structurally similar to PABA, making them ideal competitive inhibitors. Therefore, A. borkumensis YdaH may act as a drug efflux pump, capable of extruding sulfonamide antimetabolites. It is interesting to note that sulfonamides were used between the late 1930s and early 1940s to treat gonorrhoea, but the rapid emergence of strains resistant to this class of drug has resulted in its removal from the list of recommended drug therapies [27] . To determine if A. borkumensis YdaH behaves as a sulfonamide efflux pump, we transformed BL21(DE3)Δ abgT Δ pabA with pET15bΩ ydaH or pET15b and tested the susceptibility of these transformants to four different sulfonamide drugs ( Supplementary Table 2 ). Specifically, sulfamethazine was chosen because of the availability of its radioactive analogue. It is important to stress that in many instances, the expression of drug efflux pumps, including members of the resistance-nodulation-cell division [28] and multidrug and toxic compound extrusion [29] superfamilies, can have only modest changes (twofold) in bacterial susceptibility to certain antimicrobials, while more significant changes in susceptibility to other agents can be observed in the same system. We found that the BL21(DE3)Δ abgT Δ pabA cells expressing A. borkumensis YdaH were 32-fold less sensitive to sulfamethazine when compared with BL21(DE3)Δ abgT Δ pabA cells containing the empty pET15b vector. In addition, these BL21(DE3)Δ abgT Δ pabA /pET15bΩ ydaH cells were eight times more resistant to sulfanilamide when compared with the double-knockout cells transformed with the empty pET15b vector. We also found that the minimum inhibitory concentrations (MICs) of BL21(DE3)Δ abgT Δ pabA /pET15bΩ ydaH cells to sulfadiazine and sulfathiazole were both greater than eight times than those of BL21(DE3)Δ abgT Δ pabA cells carrying the empty vector pET15b. These data show that YdaH may function as a drug efflux pump, which confers resistance to a variety of sulfonamides. The binding affinities of these four sulfonamide drugs, sulfamethazine, sulfadiazine, sulfathiazole and sulfanilamide, for the YdaH transporter were then determined using isothermal titration calorimetry (ITC). The data indicate that the dissociation constants, K d s, for sulfamethazine, sulfadiazine, sulfathiazole and sulfanilamide bindings are 0.41±0.03, 7.04±0.54, 0.60±0.02 and 4.97±0.26 μM, respectively ( Supplementary Fig. 6 and Supplementary Table 3 ). These ligand-binding experiments indeed confirm that YdaH is capable of recognizing a variety of sulfonamide drugs. Mutant transporters D180A, N390, W400A, P418A, R426A, D429A and N433A expressed in BL21(DE3)Δ abgT Δ pabA were then tested for their ability to confer resistance to sulfamethazine, sulfadiazine, sulfathiazole and sulfanilamide. We found that strain BL21(DE3)Δ abgT Δ pabA carrying these YdaH mutants were more sensitive to sulfamethazine and sulfanilamide in comparison with cells expressing wild-type YdaH ( Supplementary Table 2 ). As the solubilities of sulfadiazine and sulfathiazole are ∼ 250 and 500 μg ml −1 in Luria Broth (LB) medium, we cannot determine the MICs of sulfadiazine and sulfathiazole for the BL21(DE3)Δ abgT Δ pabA /pET15bΩ ydaH cells (which are >250 and >500 μg ml −1 , respectively). Nonetheless, with the exception of the R446 variant, our data indicate that strain BL21(DE3)Δ abgT Δ pabA carrying the YdaH mutants were hypersensitive to sulfadiazine and sulfathiazole in comparison with cells expressing wild-type YdaH ( Supplementary Table 2 ). The sensitivities of BL21(DE3)Δ abgT Δ pabA cells carrying the R446 mutant were also found to be >250 and >500 μg ml −1 , respectively. These data agree with the idea that these residues may be essential for the function of A. borkumensis YdaH. To support the drug-susceptibility testing results, we measured the accumulation of radioactive sulfamethazine in BL21(DE3)Δ abgT Δ pabA cells that carried pET15bΩ ydaH or pET15b. For these experiments, we compared the accumulation of sulfamethazine over time in these cells. As shown in Fig. 5 , the results indicated a lower level of [ 3 H]-sulfamethazine accumulation in BL21(DE3)Δ abgT Δ pabA cells producing A. borkumensis YdaH compared with controlled cells harbouring the empty pET15b vector, suggesting that A. borkumensis YdaH is capable of exporting sulfamethazine from the cell. 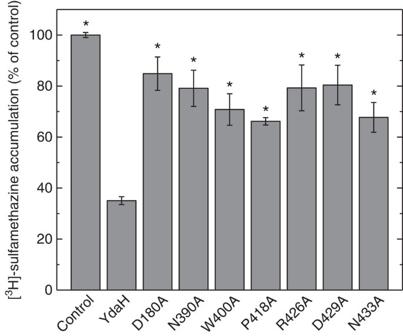Figure 5: Accumulation of radioactive sulfamethazine. E. coliBL21(DE3)ΔabgTΔpabAcells expressing YdaH show a significant decrease in [3H]-sulfamethazine accumulation when compared with cells carrying the empty vector. When transformed with plasmids expressing the mutant transporters, D180A, N390, W400A, P418A, R426A, D429A and N433A, the levels of intracellular [3H]-sulfamethazine accumulation were much higher than that of cells expressing wild-type YdaH. Error bars depict the s.d. forn=3. ‘*’ indicates values of BL21(DE3)ΔabgTΔpabA/pET15b and BL21(DE3)ΔabgTΔpabAcells expressing the mutant transporters that are significantly higher than that of BL21(DE3)ΔabgTΔpabA/pET15bΩydaHexpressing wild-type YdaH (P<0.001; Student’st-test). Figure 5: Accumulation of radioactive sulfamethazine. E. coli BL21(DE3)Δ abgT Δ pabA cells expressing YdaH show a significant decrease in [ 3 H]-sulfamethazine accumulation when compared with cells carrying the empty vector. When transformed with plasmids expressing the mutant transporters, D180A, N390, W400A, P418A, R426A, D429A and N433A, the levels of intracellular [ 3 H]-sulfamethazine accumulation were much higher than that of cells expressing wild-type YdaH. Error bars depict the s.d. for n =3. ‘*’ indicates values of BL21(DE3)Δ abgT Δ pabA /pET15b and BL21(DE3)Δ abgT Δ pabA cells expressing the mutant transporters that are significantly higher than that of BL21(DE3)Δ abgT Δ pabA /pET15bΩ ydaH expressing wild-type YdaH ( P <0.001; Student’s t -test). Full size image When transformed with plasmids expressing the mutant transporters D180A, N390A, W400A, P418A, R426A, D429A and N433A, the levels of intracellular sulfamethazine accumulation were much higher than that of cells expressing wild-type YdaH ( Fig. 5 ). Again, these data indicate that residues D180, N390, W400, P418, R426, D429 and N433 may be critical for the function of the A. borkumensis YdaH transporter. It has been suggested that members of the AbgT family use the proton-motive-force (PMF) to transport substrates across the membrane [19] . Thus, the loss of the PMF may inactivate pump activity, which results in enhanced accumulation of substrates. Accordingly, we measured the level of intracellular sulfamethazine accumulation in the presence of carbonyl cyanide m -chlorophenylhydrazone (CCCP), an uncoupler of the membrane proton gradient. After the addition of CCCP into the assay solution, the accumulation of [ 3 H]-sulfamethazine increased drastically in the YdaH-expressing cells ( Fig. 6a ), suggesting that the uncoupler CCCP was able to inhibit the function of this pump. 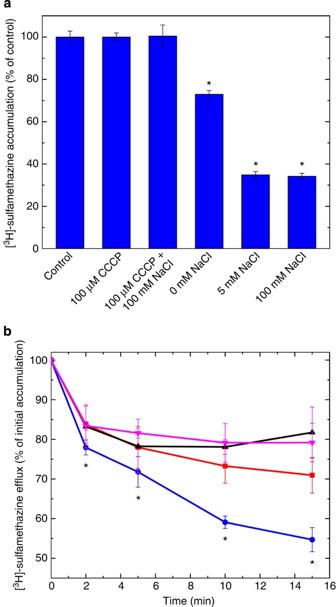Figure 6: Sodium ion enhances sulfamethazine efflux via YdaH. (a) Accumulation of radioactive sulfamethazine in BL21(DE3)ΔabgTΔpabA/pET15bΩydaHcells with difference sodium ion concentrations. Cells showed a significant decrease in [3H]-sulfamethazine accumulation in the presence of Na+. Error bars denote s.d. (n=3). ‘*’ indicates values of BL21(DE3)ΔabgTΔpabA/pET15b cells (control) that are significantly different from those of BL21(DE3)ΔabgTΔpabA/pET15bΩydaHexpressing wild-type YdaH (P<0.001; Student’st-test). (b) Efflux of radioactive sulfamethazine in BL21(DE3)ΔabgTΔpabA/pET15bΩydaHcells in the presence of sodium or potassium ions. The presence of Na+significantly enhances [3H]-sulfamethazine efflux in BL21(DE3)ΔabgTΔpabA/pET15bΩydaHcells (black, control cells with the empty vector; red, 0 mM NaCl; magenta, 5 mM KCl; blue, 5 mM NaCl). Error bars denote the s.d. (n=3). ‘*’ indicates values of radioactive counts of intracellular [3H]-sulfamethazine in BL21(DE3)ΔabgTΔpabA/pET15bΩydaHcells with 5 mM NaCl (blue) that are significantly different from those of the control (black;P<0.001; Student’st-test). Figure 6: Sodium ion enhances sulfamethazine efflux via YdaH. ( a ) Accumulation of radioactive sulfamethazine in BL21(DE3)Δ abgT Δ pabA /pET15bΩ ydaH cells with difference sodium ion concentrations. Cells showed a significant decrease in [ 3 H]-sulfamethazine accumulation in the presence of Na + . Error bars denote s.d. ( n =3). ‘*’ indicates values of BL21(DE3)Δ abgT Δ pabA /pET15b cells (control) that are significantly different from those of BL21(DE3)Δ abgT Δ pabA /pET15bΩ ydaH expressing wild-type YdaH ( P <0.001; Student’s t -test). ( b ) Efflux of radioactive sulfamethazine in BL21(DE3)Δ abgT Δ pabA /pET15bΩ ydaH cells in the presence of sodium or potassium ions. The presence of Na + significantly enhances [ 3 H]-sulfamethazine efflux in BL21(DE3)Δ abgT Δ pabA /pET15bΩ ydaH cells (black, control cells with the empty vector; red, 0 mM NaCl; magenta, 5 mM KCl; blue, 5 mM NaCl). Error bars denote the s.d. ( n =3). ‘*’ indicates values of radioactive counts of intracellular [ 3 H]-sulfamethazine in BL21(DE3)Δ abgT Δ pabA /pET15bΩ ydaH cells with 5 mM NaCl (blue) that are significantly different from those of the control (black; P <0.001; Student’s t -test). Full size image CCCP appears to inhibit the pump activity, indicating that YdaH is PMF dependent. However, it has been observed that the proton-mediated secondary transporter Salmonella typhimurium MalB is also regulated by Na + (ref. 30 ). As the crystal structure of YdaH poses the possibility that a Na + ion is bound within each subunit of this transporter, we then investigated if the presence of Na + affects intracellular drug accumulation. Specifically, we determined the accumulation level of radioactive sulfamethazine in strain BL21(DE3)Δ abgT Δ pabA /pET15bΩ ydaH in the presence of 5 or 100 mM NaCl. In both the cases, the levels of accumulation of [ 3 H]-sulfamethazine were significantly lower compared with that in the YdaH-producing strain without the addition of Na + ions ( Fig. 6a ). The results indicate that A. borkumensis YdaH functions more efficiently in the presence of Na + ions. To confirm that the presence of Na + enhances the function of the YdaH transporter, we next measured the efflux of radioactive sulfamethazine that had accumulated in strain BL21(DE3)Δ abgT Δ pabA /pET15bΩ ydaH , both in the absence and presence of Na + or K + . Cells were first loaded with [ 3 H]-sulfamethazine and CCCP was added to inhibit the pump. Thereafter, CCCP was removed and glucose was added to re-energize these cells. Cellular [ 3 H]-sulfamethazine levels were measured over time both in the absence and presence of 5 mM NaCl or KCl. As shown in Fig. 6b , the addition of Na + , but not K + , has a strong effect on sulfamethazine efflux in BL21(DE3)Δ abgT Δ pabA /pET15bΩ ydaH . In this paper, we reported the crystal structure of the A. borkumensis YdaH transporter, revealing a dimeric molecule with a fold very distinct from other families of transporters. On the basis of additional experimental data, we propose that YdaH could function as a drug efflux pump, capable of removing sulfonamide antimetabolites and mediate resistance to this class of drugs in bacterial cells. It is possible that other members of the AbgT family of transporters may serve as antimetabolite efflux pumps to protect cells against these noxious agents. Overall, our data suggest a novel mechanism for sulfonamide antimetabolite resistance in bacteria, which should be further characterized in future studies. Purification of A. borkumensis YdaH In brief, the full-length YdaH membrane protein containing a 6 × His tag at the N terminus was overproduced in E. coli BL21(DE3)Δ acrB cells, which harbours a deletion in the chromosomal acrB gene, possessing pET15bΩ ydaH . Cells were grown in 12 l of LB medium with 100 μg ml −1 ampicillin at 25 °C. When the OD 600 nm reached 0.5, the culture was treated with 0.2 mM isopropyl-β- D -thiogalactopyranoside (IPTG) to induce ydaH expression, and the cells were harvested within 15 h. The collected bacteria were resuspended in low salt buffer containing 100 mM sodium phosphate (pH 7.2), 10% glycerol, 1 mM EDTA and 1 mM phenylmethanesulfonyl fluoride (PMSF) and then disrupted with a French pressure cell. The membrane fraction was collected and washed twice with high salt buffer containing 20 mM sodium phosphate (pH 7.2), 2 M KCl, 10% glycerol, 1 mM EDTA and 1 mM PMSF and once with 20 mM HEPES-NaOH buffer (pH 7.5) containing 1 mM PMSF as described previously [31] . The membrane protein was then solubilized in 2% (w/v) n -dodecyl-β- D -maltoside (DDM). Insoluble material was removed by ultracentrifugation at 100,000 g . The extracted protein was purified with a Ni 2+ -affinity column. The purified protein was dialysed and concentrated to 20 mg ml −1 in a buffer containing 20 mM Na-HEPES (pH 7.5) and 0.05% DDM. The 6 × His tag at the N terminus was then cleaved by adding 5 U of thrombin (GE Healthcare Bio-Sciences, Pittsburgh, PA) per mg of purified YdaH at room temperature for 20 h. The protein was subsequently passed through a Ni 2+ -affinity column to remove the free 6xHis tag. A final purification step was performed using a G200 size exclusion column loaded with buffer solution containing 20 mM Na-HEPES (pH 7.5) and 0.05% DDM. The purity of the YdaH protein (>95%) was judged using 10% SDS-PAGE stained with Coomassie Brilliant Blue. The purified protein was then concentrated to 20 mg ml −1 in a buffer containing 20 mM Na-HEPES (pH 7.5) and 0.05% DDM. For 6 × His selenomethionyl-substituted (SeMet)-YdaH protein expression, a 10 ml LB broth overnight culture containing E. coli BL21(DE3) ΔacrB /pET15bΩ ydaH cells was transferred into 120 ml of LB broth containing 100 μg ml −1 ampicillin and grown at 37 °C. When the OD 600 nm value reached 1.2, cells were harvested by centrifugation at 6,000revolutions min −1 for 10 min, and then washed two times with 20 ml of M9 minimal salts solution. The cells were resuspended in 120 ml of M9 media and then transferred into a 12-l prewarmed M9 solution containing 100 μg ml −1 ampicillin. The cell culture was incubated at 25 °C with shaking. When the OD 600 nm reached 0.4, 100 mg l −1 of lysine, phenylalanine and threonine, 50 mg l −1 isoleucine, leucine and valine and 60 mg l −1 of L -selenomethionine were added. The culture was induced with 0.2 mM IPTG after 15 min. Cells were then harvested within 15 h after induction. The procedures for purifying SeMet-YdaH were identical to those of the native protein. Crystallization of YdaH Crystals of the YdaH protein were obtained using sitting-drop vapour diffusion. The YdaH crystals were grown at room temperature in 24-well plates with the following procedures. A 2-μl protein solution containing 20 mg ml −1 YdaH in 20 mM Na-HEPES (pH 7.5) and 0.05% (w/v) DDM was mixed with a 2-μl of reservoir solution containing 28% polyethylene glycol (PEG) 400, 0.1 M sodium acetate (pH 5.0), 0.05 M magnesium acetate, 3% glycerol and 2% (w/v) n -octyl-β- D -glucoside. The resultant mixture was equilibrated against 500 μl of the reservoir solution at 25 °C. The crystallization conditions for SeMet-YdaH were the same as those for the native YdaH protein. Crystals of both YdaH and SeMet-YdaH grew to a full size in the drops within a month. Typically, the dimensions of the crystals were 0.2 × 0.2 × 0.2 mm. Cryoprotection was achieved by raising the PEG 400 concentration to 32% in a single step. Crystals of the tungsten cluster derivative were prepared by incubating the crystals of YdaH in solution containing 32% PEG 400, 0.1 M sodium acetate (pH 5.0), 0.05 M magnesium acetate, 3% glycerol and 2% (w/v) n -octyl-β- D -glucoside, 0.05% (w/v) DDM and 0.5 mM Na 9 [β-SiW 9 O 34 H]·23H 2 O for 4 h at 25 °C. Data collection and structural determination All diffraction data were collected at 100 K at beamline 24ID-C located at the Advanced Photon Source, using a Platus 6M detector. Diffraction data were processed using DENZO and scaled using SCALEPACK [32] . Crystals of YdaH belonged to space group P 2 1 ( Table 1 ). On the basis of the molecular weight of YdaH (51.6 kDa), four molecules per asymmetric unit with a solvent content of 73.4% were expected. The heavy-atom derivative ([β-SiW 9 O 34 H] 9− cluster) [33] was isomorphous with the native crystal ( Table 1 ). Six heavy-atom sites for the tungsten derivative were identified using SHELXC and SHELXD [34] as implemented in the HKL2MAP package [35] . These heavy-atom sites were refined using the programme MLPHARE [36] , [37] . The resulting phases were subjected to density modification and fourfold NCS averaging by RESOLVE [38] using the native structure factor amplitudes. Density-modified phases allowed us to visualize the helical structural features of the molecule. The initial model was built manually using Coot [39] . The SeMet data were then used to help determine the 4.10-Å-resolution structure of YdaH by molecular replacement with single-wavelength anomalous diffraction using the programme Phaser [40] . The manually built model was used as initial search model. The full-length YdaH protein consists of 11 methionine residues and all of these 11 selenium sites were identified in each protomer of the protein (44 total selenium sites in the asymmetric unit). These phases were then improved by NCS averaging with density modification using the programme RESOLVE [38] . The resulting phases were of excellent quality, which enabled us to trace of most of the molecule. After tracing the initial model manually using the programme Coot [39] , the model was refined using PHENIX [41] leaving 5% of the reflections in Free-R set. Iterations of refinement using PHENIX [41] and CNS [42] and model building in Coot [39] lead to the 4.10-Å-resolution structural model of the YdaH transporter. This structure was then used to refine against the 2.96-Å-resolution data using PHENIX [41] as described above. Iterations of refinement using PHENIX [41] and CNS [42] and model building in Coot [39] lead to the current 2.96-Å-resolution model with excellent geometrical characteristics ( Table 1 ). Gel filtration A protein liquid chromatography Superdex 200 16/60 column (GE Healthcare, Pittsburgh, PA) with a mobile phase containing 20 mM Na-HEPES (pH 7.5) and 0.05% (w/v) DDM was used in the gel filtration experiments. Blue dextran (Sigma-Aldrich, St Louis, MO) was used to determine the column void volume. As there are no commercially available membrane protein markers, we used the well-characterized N. gonorrhoeae NorM multidrug efflux pump [43] , [44] (which exists as a monomer in solution with the monomeric molecular weight equals 50.6 kDa) and E. coli CusC outer membrane channel [45] , [46] (which exists as a trimer in solution with the trimeric molecular weight equals 147.7 kDa) as standards. The experiments were repeated for three times. Gel filtration suggested an average molecular weight of 107.0±8.8 kDa for the YdaH transporter ( Supplementary Fig. 4 ). This value is in good agreement with the theoretical value of 105.6 kDa for two YdaH protomers. Construction of the double knockout strain The double-knockout E. coli strain BL21(DE3)Δ abgT Δ pabA was produced from the BL21(DE3) strain using an RED disruption system as described by Datsenko and Wanner [47] . The Δ abgT::kan cassette, which was used to replace the chromosomal abgT gene, was produced by PCR, and then introduced into pKD46/BL21(DE3) by electroporation. The knockout BL21(DE3)Δ abgT::kan strain was selected on LB plate containing 30 μg ml −1 kanamycin, and verified by PCR. The kanamycin-resistant gene was then released to generate the BL21(DE3)Δ abgT knockout strain. The deletion of pabA from BL21(DE3)Δ abgT was done using similar procedures as described above to generate the final BL21(DE3)Δ abgT Δ pabA double-knockout strain. Site-directed mutagenesis Site-directed point mutations on residues D180, N390, W400, P418, R426, D429 and N433, which are expected to be critical for the function of the YdaH transporter, were performed to generate the single point mutants D180A, N390A, W400A, P418A, R426A, D429A and N433A. The primers used for these mutations are listed in Supplementary Table 2 . All oligonucleotides were purchased from (Integrated DNA Technologies Inc., Coralville, IA) in a salt-free grade. Accumulation assays of PABA In brief, E. coli BL21(DE3)Δ abgT Δ pabA carrying pET15bΩ ydaH or pET15b were grown in LB broth with 100 μg ml −1 ampicillin at 37 °C. When the OD 600 nm reached 0.5, the culture was treated with 0.2 mM IPTG to induce ydaH expression, and cells were harvested within 2 h. Cells were washed twice with buffer containing 50 mM potassium phosphate (pH 7.5), twice with buffer containing 100 mM Tris-HCl (pH 7.5) and 5 mM NaCl, and then suspended in the same buffer to OD 600 nm of 15. [ 3 H]-PABA (Moravek Biochemicals, Brea, CA) was then added to a final concentration of 0.3 μM. The specific activity of [ 3 H]-PABA is 30.4 Ci mmol −1 . Samples of 100 μl were taken at intervals, applied directly to prewetted glass-fibre filters, and washed twice with 5-ml aliquots of the same buffer; 0.5-μm glass-fiber filters (MFS, Dubbin, CA) were used with a filter apparatus. Filters were then incubated for 30 min in scintillation fluid (ScintiVerse BD) and counted with a Packard Tri-Carb 1600TR liquid scintillation counter (Perkin Elmer, Waltham, MA). For [ 3 H]-PABA accumulations in cells expressing the YdaH mutants, the procedures for sample preparation were the same as above. Cells were incubated with 0.3 μM [ 3 H]-PABA for 15 min, applied directly to prewetted glass-fibre filters and washed immediately twice with 5-ml aliquots of the same buffer. Filters were then incubated for 30 min in scintillation fluid (ScintiVerse BD) and counted with a Packard Tri-Carb 1600TR liquid scintillation counter (Perkin Elmer, Waltham, MA). Assays of folic acid The concentration of folic acid in the double-knockout BL21(DE3)Δ abgT Δ pabA strain transformed with pET15bΩ ydaH or pET15b was measured using Lactobacillus casei based on the microbiological procedure of Wilson and Horne [25] . The concentrations of folic acid in BL21(DE3)Δ abgT Δ pabA expressing the mutant transporters were measured using the same procedures. Drug-susceptibility assays The susceptibilities to sulfamethazine, sulfadiazine, sulfathiazole and sulfanilamide of E. coli BL21(DE3)Δ abgT Δ pabA harbouring pET15bΩ ydaH expressing the wild-type or mutant transporters, or the pET15b empty vector were tested on agar plates. Cells were grown in LB medium with 100 μg ml −1 ampicillin at 37 °C. When the OD 600 nm reached 0.5, the cultures were induced with 0.2 mM IPTG and harvested for 2 h after induction. The minimum growth inhibitory concentrations (MICs) of sulfamethazine and sulfanilamide for E. coli BL21(DE3)Δ abgT Δ pabA (incoculum, 500 cells ml −1 ) harbouring these vectors were then determined using LB agar containing 50 μg ml −1 ampicillin, 0.1 mM IPTG and different concentrations of sulfamethazine and sulfanilamide, respectively. Isothermal titration calorimetry We used ITC to examine the binding of sulfamethazine, sulfadiazine, sulfathiazole or sulfanilamide to the purified YdaH transporter. Measurements were performed on a VP-Microcalorimeter (MicroCal, Northampton, MA) at 25 °C. Before titration, the protein was thoroughly dialysed against buffer containing 20 mM Tris-HCl pH 7.5, 50 mM NaCl and 0.03% DDM. The protein concentration was determined using the Bradford assay. The protein sample was then adjusted to a final concentration of 20 μM. Ligand solution consisting of 0.4 mM sulfamethazine, sulfadiazine, sulfathiazole or sulfanilamide in 20 mM Tris-HCl pH 7.5, 50 mM NaCl and 0.03% DDM was prepared as the titrant. The protein and ligand samples were degassed before they were loaded into the cell and syringe. Binding experiments were carried out with the protein solution (1.5 ml) in the cell and the ligand as the injectant. Ten μl injections of the ligand solution were used for data collection. Injections occurred at intervals of 300 s, and the duration time of each injection was 20 s. Heat transfer (μcal s −1 ) was measured as a function of elapsed time (s). The mean enthalpies measured from injection of the ligand in the buffer were subtracted from raw titration data before data analysis with ORIGIN software (MicroCal). Titration curves were fitted by a non-linear least-squares method to a function for the binding of a ligand to a macromolecule. Non-linear regression fitting to the binding isotherm provided us with the equilibrium binding constant ( K a =1/ K d ) and enthalpy of binding (Δ H ). On the basis of the values of K A , the change in free energy (Δ G ) and entropy (Δ S ) were calculated with the equation: Δ G =−RT ln K a =Δ H−T Δ S , where T is 273 K and R is 1.9872, cal K −1 per mol. Calorimetry trials were also carried out in the absence of YdaH in the same experimental conditions. No change in heat was observed in the injections throughout the experiment. Accumulation assays of sulfamethazine The procedures for [ 3 H]-sulfamethazine accumulation were the same as those for [ 3 H]-PABA accumulation. The specific activity of [ 3 H]-sulfamethazine is 34.5 Ci mmol −1 . Cells were incubated with 75 nM [ 3 H]-sulfamethazine (Moravek Biochemicals, Brea, CA) for 15 min, applied directly to prewetted glass-fibre filters and washed immediately twice with 5-ml aliquots of the same buffer. Filters were then incubated for 30 min in scintillation fluid (ScintiVerse BD) and counted with a Packard Tri-Carb 1600TR liquid scintillation counter (Perkin Elmer, Waltham, MA). For the Na + -dependent experiments, cells were incubated with 75 nM [ 3 H]-sulfamethazine in the presence of NaCl (0, 5 or 100 mM) for 15 min, then applied directly to prewetted glass-fibre filters and washed immediately twice with 5-ml aliquots of buffer containing 100 mM Tris-HCl (pH 7.5) and 0, 5 or 100 mM NaCl. Efflux assays of sulfamethazine E. coli BL21(DE3)Δ abgT Δ pabA carrying pET15bΩ ydaH or pET15b were grown in LB broth with 100 μg ml −1 ampicillin at 37 °C. When the OD 600 nm reached 0.5, the culture was induced with 0.2 mM IPTG and the cells were harvested within 2 h. Cells were washed twice with buffer containing 50 mM potassium phosphate (pH 7.5), twice with buffer containing 100 mM Tris-HCl (pH 7.5) and then suspended in the same buffer to OD 600 nm of 15. CCCP was added to the cell suspension at a final concentration of 100 μM. Cells were then incubated for 10 min, pelleted, washed twice and resuspended in the same buffer to OD 600 nm of 10. [ 3 H]-sulfamethazine was then added to a final concentration of 37 nM. Cells were incubated for 15 min, and a final concentration of 0.2% glucose was then added to the cell suspension. When needed, a final concentration of 5 mM NaCl or KCl was also added at the same time. At various time points, samples of 100 μl were applied directly to prewetted glass-fibre filters, and washed twice with 5-ml aliquots of buffer containing 100 mM Tris-HCl (pH 7.5). Filters were then incubated for 30 min in scintillation fluid (ScintiVerse BD) and counted with a Packard Tri-Carb 1600TR liquid scintillation counter (Perkin Elmer, Waltham, MA). How to cite this article: Bolla, J.R. et al. Crystal structure of the Alcanivorax borkumensis YdaH transporter reveals an unusual topology. Nat. Commun. 6:6874 doi: 10.1038/ncomms7874 (2015). Accession code: Atomic coordinates and structure factors for the structure of YdaH have been deposited at the RCSB Protein Data Bank with an accession code 4R0C .